Coherent two-dimensional photocurrent spectroscopy in a PbS quantum dot photocell Recently there has been growing interest in the role of coherence in electronic dynamics. Coherent multidimensional spectroscopy has been used to reveal coherent phenomena in numerous material systems. Here we utilize a recent implementation of coherent multidimensional spectroscopy—two-dimensional photocurrent spectroscopy—in which we detect the photocurrent from a PbS quantum dot photocell resulting from its interactions with a sequence of four ultrafast laser pulses. We observe sub-picosecond evolution of two-dimensional spectra consistent with multiple exciton generation. Moreover, a comparison with two-dimensional fluorescence spectra of the quantum dots demonstrates the potential of two-dimensional photocurrent spectroscopy to elucidate detailed origins of photocurrent generating electronic state coherence pathways. Since the measurement is based on detecting the photocell current in situ , the method is well suited to study the fundamental ultrafast processes that affect the function of the device. This opens new avenues to investigate and implement coherent optimization strategies directly within devices. The optical properties of quantum dots (QDs) are strongly influenced by the dynamics of electronically excited electron–hole pairs (called excitons), which are generated by the absorption of a photon from an external optical field. More than one exciton can be simultaneously excited within a QD, either by increasing the optical field strength (that is, the photon density) [1] or by increasing its frequency (the photon energy) [2] , [3] . In the former process, a sequential absorption of m photons leads to the creation of m excitons. In the latter process, which is called multiple exciton generation (MEG), the number of excitons created exceeds the number of photons absorbed [4] . MEG is a transient non-linear phenomenon in which many-body interactions transform a single high-energy excitation into two or more low-energy electron–hole pairs. In general, many-body effects can lead to time-dependent shifts of the electronic resonance frequency of the QDs due to the dynamics of local fields, which are themselves induced by the presence of excitons [5] , [6] . Such effects in nanoconfined systems are readily observed using non-linear spectroscopic methods. In particular, two-dimensional electronic spectroscopy (2DES) can be used to study many-body effects in semiconductor nanoparticles, quantum wells and atomic vapours [7] , [8] , [9] . In conventional 2DES [10] , [11] , [12] , [13] , a coherent optical signal results from three non-collinear ultrafast laser pulses, which interact resonantly with a material system. The signal is detected in the wavevector-matched direction as a function of interpulse delay, and Fourier transformed with respect to the appropriate time variables to construct a 2D optical spectrum. Such 2D spectroscopic techniques provide complete information about field–matter interaction pathways that contribute to the third-order optical response of the system [11] , [13] , [14] . These pathways, which are termed ground state bleach (GSB), stimulated emission (SE) and excited state absorption (ESA) involve interaction with three laser pulses. The pathways lead to a non-linear polarization that emits in the signal direction as the fourth system-field interaction. GSB, SE and ESA pathways are grouped into rephasing (RP) and non-rephasing (NRP) pathways according to their phase-matching conditions. An alternative approach to 2D spectroscopy uses a sequence of four collinear laser pulses (see Fig. 1a ), in which case the fourth pulse drives the final field–system interaction. The resulting excited-state populations are detected by monitoring an incoherent ‘action signal,’ such as fluorescence or photocurrent, which depends on the state-specific quantum yield of the process generating the signal. This is the basis of 2D fluorescence spectroscopy (2DFS) that was previously developed by one of us to measure the 2D spectra of fluorescent systems [15] . 2DFS has been used to study the conformations and excited-state energy transfer of exciton-coupled molecular dimers in biological membranes and in nucleic acids [16] , [17] , [18] , [19] . 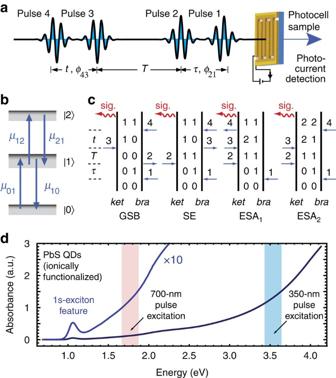Figure 1: Schematic 2DPS experimental setup, electronic coherence pathways and sample absorption spectrum. (a) Phase-modulation 2DPS pulse sequence and detection scheme. (b) Energy level diagram indicating state labels and resonant transitions induced by pulse interactions. (c) Double-sided Feynman diagrams indicating the four possible non-linear electronic transition pathways that are detected by the 2DPS experiment. For brevity, only the RP pathways are shown. There is one GSB, one SE, and two excited state absorption (ESA1(2)) pathways. The 2DPS signal is given by=GSB+SE+ESA1−Γ·ESA1, where Γ≥0 represents the photocurrent quantum yield associated with excitons created on state-|2› relative to the quantum yield associated with excitons created on state-|1›. (d) Absorption spectrum, collected in D2O, of the sodium 2,3-DT-capped PbS nanoparticles used for the 2DPS measurements. The excitation energy conditions using 700 and 350 nm light are shown relative to the band edge feature. Figure 1: Schematic 2DPS experimental setup, electronic coherence pathways and sample absorption spectrum. ( a ) Phase-modulation 2DPS pulse sequence and detection scheme. ( b ) Energy level diagram indicating state labels and resonant transitions induced by pulse interactions. ( c ) Double-sided Feynman diagrams indicating the four possible non-linear electronic transition pathways that are detected by the 2DPS experiment. For brevity, only the RP pathways are shown. There is one GSB, one SE, and two excited state absorption (ESA 1(2) ) pathways. The 2DPS signal is given by =GSB+SE+ESA 1 −Γ·ESA 1 , where Γ≥0 represents the photocurrent quantum yield associated with excitons created on state-|2› relative to the quantum yield associated with excitons created on state-|1›. ( d ) Absorption spectrum, collected in D 2 O, of the sodium 2,3-DT-capped PbS nanoparticles used for the 2DPS measurements. The excitation energy conditions using 700 and 350 nm light are shown relative to the band edge feature. Full size image In this work, we perform a variation of 2DFS that monitors the non-linear photocurrent signal induced by a four-pulse laser sequence. This technique, which we call the 2D photocurrent spectroscopy (2DPS), utilizes acousto-optic phase modulation of the exciting laser pulse train in combination with phase-synchronous detection of the ensuing photocurrent signal. This highly sensitive approach is ideally suited to distinguish between the excitation pathways that lead to MEG, and those that do not, since the action signal is a quantum yield-dependent function of the number of excitons generated within the photocell. Recently, Cundiff and co-workers [20] demonstrated photocurrent-detected 2DES in a semiconductor nanostructure using this same approach. Here we perform 2DPS on a PbS colloidal QD photocell using two different laser excitation energies, both of which are well above the semiconductor band edge. We find that the electronic coherence pathways responsible for photocurrent generation reflect very different local field-induced dynamics under low- and high-energy excitation conditions. Under high-energy conditions, the 2DPS lineshape undergoes sub-picosecond evolution from absorptive to dispersive character, which is due to a time-dependent shift of the resonant transition energies. We interpret these data in terms of the manifestation of MEG on the picosecond timescale. In contrast, we observe no field-induced dynamics under low-energy excitation conditions. In addition, we compare photocurrent and fluorescence detected 2D lineshapes, which exhibit qualitatively different character. These experiments demonstrate that our approach can be used to separately determine the coherence pathways responsible for photocurrent generation versus fluorescence. Two-dimensional action spectroscopy In a phase-modulation four-pulse experiment, an incoherent ‘action signal’ (that is, fluorescence or photocurrent) is monitored as a function of the time delays between pulses 1 and 2 (called the coherence time, τ ) and between pulses 3 and 4 (called the detection time, t , see Fig. 1a ). The time delay between pulses 2 and 3 is called the population time, T . The effect of each pulse is to transfer amplitude between ground-, first- and second-excited states, which we designate as states-|0›, |1› and |2›, respectively (see Fig. 1b ). The evolution of coherences and populations during the intervals τ , T and t , and their influence on the final populations of excitons that give rise to the photocurrent signal, leads to the 2D response function S ( τ , T , t ). Fourier transformation of the response function with respect to the variables τ and t yields the 2D spectrum (refs 16 , 17 ). These spectra are recorded as a parametric function of the variable T , and changes in the 2D spectral line shape provide detailed information about excited state processes that occur on ultrafast timescales. The 2D optical spectrum is composed of three types of excitation pathways that are designated as GSB, SE and ESA, and which are described using double-sided Feynman diagrams (see Fig. 1c ) [16] , [17] . It follows from time-dependent perturbation theory that the sign corresponding to each excitation pathway depends on whether there is an even or an odd number of field–matter interactions appearing on the bra side of the double-sided Feynman diagrams [21] . There is one GSB and one SE pathway that each contribute to the signal with the same sign and produce population of excitons in state-|1›, while there are two different ESA pathways that each contribute with opposite signs. In the first ESA pathway (ESA 1 ), the final population of excitons (after the passage of all four pulses) resides in state-|1›, which is the same as that just before the interaction with the third pulse. In the second ESA pathway (ESA 2 ), the final population of excitons resides in state-|2› with a higher energy than that of state-|1›. The first ESA pathway contributes with the same sign as the GSB and SE pathways, while the second ESA pathway contributes with opposite sign. These four excitation pathways contribute to the cumulative photocurrent signal according to GSB+SE+ESA 1 −ESA 2 , where ESA 2 =Γ·ESA 1 and Γ≥0 represents the photocurrent quantum yield associated with excitons created on state-|2› relative to the quantum yield associated with excitons created on state-|1›. We note that in previous fluorescence-detected 2D experiments performed on condensed phase molecular systems [16] , [17] , [18] , [19] , we typically observed the value of Γ<1, indicating that the fluorescence quantum yield from high-lying excited states is small (due to radiationless deactivation processes) in comparison with the fluorescence yield from low-lying excited states. For photocurrent-detected 2D experiments, we anticipate that the value of Γ may be much larger than for the corresponding fluorescence case (that is, Γ>1), since we expect the photocurrent quantum yield to be enhanced for high-lying excited states in comparison to low-lying states. Many-body effects and excitation induced shifts in QDs The optical response of QDs can be described using the semiconductor Bloch equations. In this description, local fields induced by the many-body effects resulting from pre-existing electron–hole pairs lead to renormalization of the energy and electronic dephasing of the optical transition [5] , [7] . This change of the transition energy is referred to as an excitation-induced shift (EIS), and the dephasing results in broadening of the optical line shape. For experiments that use photon energies close to the band edge, it has been shown that many-body correlation effects beyond the mean field approximation must be considered to describe the details of the 2D spectra [22] . In our current work, we used photon energies at 1.6 E g and 3.2 E g that are well above the band edge (see Fig. 1d ), so that a continuum of states is excited. Under these conditions, it is justified to invoke the EIS even though the derivation of the semiconductor Bloch equations is based on the mean field approximation. The hot electron population created by the first two laser pulses is expected to rapidly relax from its resonance condition with the laser, such that the SE contribution to the cumulative signal will be negligible for T >0. Similarly, the local fields induced by the many-body effects are not expected to influence the evolution of the ground-state energy, and thus the GSB contribution to the cumulative signal is expected to be independent of the EIS [23] . The most significant time-dependent manifestations of the many-body effects are expected to occur in the ESA signal contributions, where the EIS will lead to a vertical displacement of the 2D bands. In the event that the photocurrent quantum yield from state-|2› is high (that is, Γ>1), the combined effects of the different excitation pathways will lead to a partial cancellation of positive and negative terms that are vertically offset from one another within the 2D spectrum, thus leading to an apparent dispersive line shape. In Fig. 2 , we present 2DPS RP spectra that were recorded as a function of the population delay T for a PbS colloidal QD photocell in which the laser excitation spectrum was centred at ~700 nm (14,286 cm −1 =1.8 eV). The QDs used in these samples have a band gap E g ~1.1 eV and are capped with the short-chain dithiol ligand sodium 2,3-dimercaptopropanesulfonate (DT). The laser intensity was set to a relatively low value (~10 8 photons cm −2 per pulse) to ensure that no more than one photon was absorbed per QD after the interaction with the first two pulses. Although biexcitons are generated in the second of the two ESA pathways, the 2D spectral line shape exhibits primarily absorptive character. Thus, under these excitation conditions (~1.6 E g ), we did not observe evidence of a significant EIS. 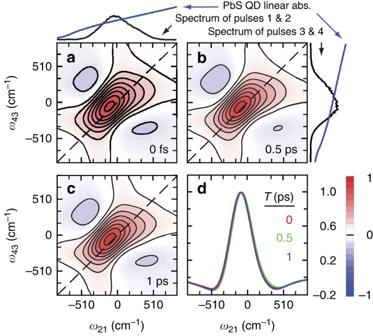Figure 2: 2DPS measurements performed under low-energy excitation conditions. RP 2DPS data taken from a PbS QD photocell. The pulse excitation wavelength was centred at 700 nm (=14,286 cm−1=1.8 eV≃1.6Eg). 2D spectra are shown for the population timesT=0 fs (a), 500 fs (b) and 1 ps (c). The axes are rescaled to show the line shape relative to the peak laser pulse energy. Laser pulse and QD absorption spectra are shown, as indicated. The 2D spectra exhibit a predominantly absorptive line shape, which is independent of the population periodT. (d) Cross-sections of the 2D line shape along the antidiagonal direction for each value ofT. Figure 2: 2DPS measurements performed under low-energy excitation conditions. RP 2DPS data taken from a PbS QD photocell. The pulse excitation wavelength was centred at 700 nm (=14,286 cm −1 =1.8 eV ≃ 1.6 E g ). 2D spectra are shown for the population times T =0 fs ( a ), 500 fs ( b ) and 1 ps ( c ). The axes are rescaled to show the line shape relative to the peak laser pulse energy. Laser pulse and QD absorption spectra are shown, as indicated. The 2D spectra exhibit a predominantly absorptive line shape, which is independent of the population period T . ( d ) Cross-sections of the 2D line shape along the antidiagonal direction for each value of T . Full size image We next examined the behaviour of the 2DPS line shape under conditions of relatively high excitation energy. Efficient MEG is known to occur in PbS QDs when the excitation energy is greater than ~3 E g (ref. 24 ). To create multiple-exciton states in the PbS QDs via MEG, we performed 2DPS experiments on the same photocells as described above, but using laser pulses with center wavelength set to 351 nm (28,490 cm −1 =3.5 eV ≃ 3.2 E g ), as described previously [18] . In Fig. 3 , we show 2DPS RP data recorded as a function of the population delay T . At zero population delay ( T =0, see Fig. 3a ), the 2D line shape appeared primarily absorptive (dominant positive feature) with peak resonance shifted below the diagonal line. As the population delay was increased to T =500 fs and T =1 ps, the 2D line shape exhibited both positive and negative features of comparable magnitude, which were separated by a nodal line parallel to the diagonal (see Fig. 3b,c ). The 2D line shape appeared to undergo a qualitative change from absorptive to dispersive character due to EIS. 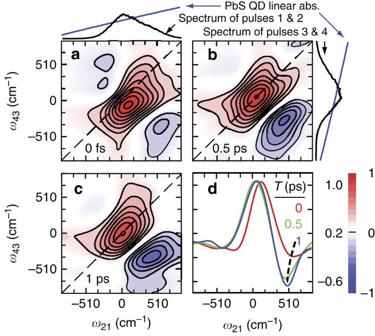Figure 3: 2DPS measurements performed under high-energy excitation conditions. RP 2DPS data taken from the same PbS QD photocell as described inFig. 2above. The sample was excited using light tuned to 351 nm (28,490 cm−1=3.5 eV≃3.2Eg). 2D spectra are shown for the population timesT=0 fs (a), 500 fs (b) and 1 ps (c). The axes are rescaled relative to the peak laser energy. Laser pulse and QD absorption spectra are shown, as indicated. The time dependence of the 2D line shape reflects the MEG arising from a high-energy exciton (see text). (d) Cross-sections of the 2D spectrum in the direction of the antidiagonal line. The curved dashed arrow indicates the formation of a dispersive lineshape in time. This evolution of the 2D line shape is consistent with the formation of multiple excitons on the sub-picosecond timescale. Figure 3: 2DPS measurements performed under high-energy excitation conditions. RP 2DPS data taken from the same PbS QD photocell as described in Fig. 2 above. The sample was excited using light tuned to 351 nm (28,490 cm −1 =3.5 eV ≃ 3.2 E g ). 2D spectra are shown for the population times T =0 fs ( a ), 500 fs ( b ) and 1 ps ( c ). The axes are rescaled relative to the peak laser energy. Laser pulse and QD absorption spectra are shown, as indicated. The time dependence of the 2D line shape reflects the MEG arising from a high-energy exciton (see text). ( d ) Cross-sections of the 2D spectrum in the direction of the antidiagonal line. The curved dashed arrow indicates the formation of a dispersive lineshape in time. This evolution of the 2D line shape is consistent with the formation of multiple excitons on the sub-picosecond timescale. Full size image In recent work, spectral shifts were observed in time-resolved pump-probe spectroscopy of PbS QDs when the dynamics were probed close to the band edge [25] . These shifts appear instantaneously after the excitation of the QDs and subsequently decay on the relaxation timescale characteristic of hot carriers. They were thus interpreted in terms of the transient Stark effect imposed by a hot electron–hole pair. The shifts we observe in our 2DPS measurements, which were carried out at energies high above the bandgap, are not instantaneous. Rather, the EIS appears over time for the case of 351 nm excitation, but not for 700 nm excitation. Hence, our results cannot be explained in terms of the transient Stark effect. The EIS induced by many-body effects is enhanced with increasing exciton density. We therefore interpret the appearance of the EIS for the case of high excitation energy as evidence for the formation of multiple excitons within the PbS QDs. Our results can provide new insights towards understanding the mechanism of MEG. Although MEG has been inferred by monitoring the Auger relaxation of multiple excitons long after their formation [4] , [24] , our 2DPS approach provides a means to directly observe the sub-picosecond MEG process in real time. The 2DPS line shape takes on dispersive characteristics within 500 fs, which persists at longer times ( Fig. 3d ). In one possible model for MEG, an initially created exciton undergoes adiabatic passage to mix with multiple exciton states [26] . An alternative model predicts an instantaneous, coherently coupled process of MEG [27] . Our results support the former model, in which multiple excitons are generated on sub-picosecond timescales through a relatively inefficient and dissipative process. In Fig. 4 , we present a proposed mechanism for the two different ESA pathways (ESA 1 and ESA 2 ) that contribute to the 2DPS signal for experiments using visible and ultraviolet light excitation. As described above, these two pathways contribute to the cumulative 2DPS signal with opposite signs and different weights, depending on the photocurrent quantum yields of the final state exciton populations. For the case of visible light experiments (see Fig. 4a,b ), the effect of the first two laser pulses is to create population within the one-exciton state, which subsequently undergoes relaxation during the time interval T . This one-exciton state does not lead to an EIS. Moreover, for the ESA 1 pathway, the one-exciton state population is unaltered by the passage of the final two laser pulses. For the second pathway (ESA 2 ), the effect of the final two laser pulses is to create population in the two-exciton state. Each excitation pathway leads to charge separation and, depending on the relative values of state-specific charge-carrier quantum yields, the generation of the photocurrent signal. The initial creation of the exciton, its relaxation during the period T and the subsequent excitation of the biexciton is depicted in Fig. 4b using a valence-conduction state diagram. 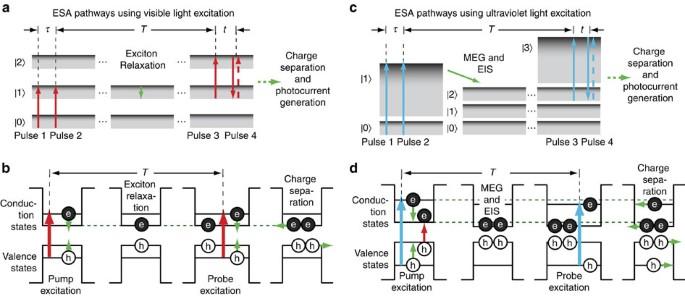Figure 4: Proposed mechanism for photocurrent generation observed in 2DPS experiments. The two excited-state absorption pathways, ESA1and ESA2, are shown for both visible (a,b) and ultraviolet (c,d) light excitation. For the case of visible excitation, the first pathway (ESA1) leads to the creation of a single exciton after the passage of the fourth laser pulse (shown inaas a solid downward red arrow that creates population on state-|1›). In the second pathway (ESA2), the fourth pulse (shown as a dashed upward red arrow) creates population on the two-exciton state-|2›. Inb, we show the valence-conduction states and exciton populations involved in the ESA2pathway. For the case of ultraviolet excitation, the initially created exciton occupies a sufficiently high-energy state so that its subsequent relaxation leads to MEG and an EIS. In the first pathway (ESA1), the population on the two-exciton state remains after the passage of the fourth laser pulse (shown incas a solid downward blue arrow), while in the second pathway (ESA2) an additional exciton is generated due to the passage of the fourth laser pulse (shown as a dashed upward blue arrow). Ind, we show the valence-conduction states involved in the ESA2pathway. Figure 4: Proposed mechanism for photocurrent generation observed in 2DPS experiments. The two excited-state absorption pathways, ESA 1 and ESA 2 , are shown for both visible ( a , b ) and ultraviolet ( c , d ) light excitation. For the case of visible excitation, the first pathway (ESA 1 ) leads to the creation of a single exciton after the passage of the fourth laser pulse (shown in a as a solid downward red arrow that creates population on state-|1›). In the second pathway (ESA 2 ), the fourth pulse (shown as a dashed upward red arrow) creates population on the two-exciton state-|2›. In b , we show the valence-conduction states and exciton populations involved in the ESA 2 pathway. For the case of ultraviolet excitation, the initially created exciton occupies a sufficiently high-energy state so that its subsequent relaxation leads to MEG and an EIS. In the first pathway (ESA 1 ), the population on the two-exciton state remains after the passage of the fourth laser pulse (shown in c as a solid downward blue arrow), while in the second pathway (ESA 2 ) an additional exciton is generated due to the passage of the fourth laser pulse (shown as a dashed upward blue arrow). In d , we show the valence-conduction states involved in the ESA 2 pathway. Full size image For experiments using ultraviolet laser pulses (see Fig. 4c,d ), the initially created exciton has an energy ~3.2 E g . The energy released during the sub-picosecond relaxation of this high-energy state can be used to promote an additional low-energy exciton, thus generating a two-exciton state during the time interval T . The Coulomb interactions between multiple excitons gives rise to an EIS, which is depicted as a lowering of the energy of all excited states. For the case of the first pathway (ESA 1 ), the photocurrent signal is generated from the charge separation of the biexciton that is created through the MEG process. For the second ESA 2 pathway, an additional high-energy exciton is generated by the action of the final two laser pulses. In this case, the photocurrent signal is generated by charge separation of both a two-exciton and an additional high-energy exciton state. A valence-conduction state diagram that depicts this latter process is shown in Fig. 4d . We have used the method of 2DPS to measure the non-linear response function of a PbS photocell. We note that many-body effects such as MEG can influence the appearance of the 2D spectrum in different ways, depending on the nature of the detection observable. To illustrate this point, we compared the two methods of photocurrent- and fluorescence-detected 2D spectroscopy carried out on PbS QDs using 351-nm pulse excitation. For this purpose, we performed the 2DFS experiments on a suspension of PbS QDs in hexane with bandgap E g =1.1 eV, in which the colloidal particles were capped with oleic acid (OLA) ligands. Although these two types of PbS samples should have different photophysical properties, both are expected to undergo MEG on excitation using 351 nm light. In Fig. 5 , we compare the real part of the 2D total correlation spectra (that is, the sum of the RP and NRP spectra) for the photocell and the colloidal suspension samples with population time T =1 ps. As previously described, the photocurrent-detected 2D spectrum exhibits a dispersive line shape under these conditions ( Fig. 5a ). However, the fluorescence-detected spectrum appears primarily absorptive ( Fig. 5b ). This result can be understood in terms of differences between photocurrent and fluorescence quantum yields associated with the final populations of high- and low-lying exciton states. 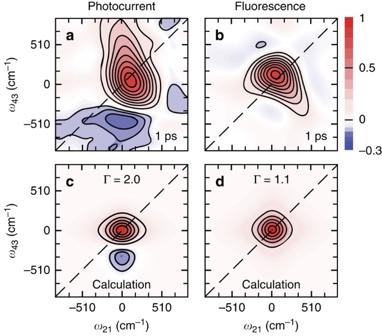Figure 5: Comparison between photocurrent and fluorescence detected 2D action spectra of PbS QDs. Real part of the 2D total correlation spectra as measured by photocurrent detection (a) and fluorescence-detection (b). Both spectra ina,bare taken with population timeT=1 ps. The dispersive 2D line shape obtained inais a consequence of the EIS caused by MEG in the PbS QDs. The predominantly absorptive signal observed inbindicates that the EIS under similar illumination conditions does not contribute significantly to fluorescence from PbS QDs in solution. The qualitative form of the 2D line shape in each case is readily reproduced from computer simulations (c,d), where the value Γ=2 corresponds to the case in which the EIS has a pronounced effect on the photocurrent-detected 2D action spectrum, while the value Γ=1.1 corresponds to the case in which the EIS has only a minor effect on the fluorescence-detected 2D action spectrum. For these simulations, the value of the EIS was assumed to be 500 cm−1. Figure 5: Comparison between photocurrent and fluorescence detected 2D action spectra of PbS QDs. Real part of the 2D total correlation spectra as measured by photocurrent detection ( a ) and fluorescence-detection ( b ). Both spectra in a , b are taken with population time T =1 ps. The dispersive 2D line shape obtained in a is a consequence of the EIS caused by MEG in the PbS QDs. The predominantly absorptive signal observed in b indicates that the EIS under similar illumination conditions does not contribute significantly to fluorescence from PbS QDs in solution. The qualitative form of the 2D line shape in each case is readily reproduced from computer simulations ( c , d ), where the value Γ=2 corresponds to the case in which the EIS has a pronounced effect on the photocurrent-detected 2D action spectrum, while the value Γ=1.1 corresponds to the case in which the EIS has only a minor effect on the fluorescence-detected 2D action spectrum. For these simulations, the value of the EIS was assumed to be 500 cm −1 . Full size image Multiple excitons in QDs do not efficiently contribute to fluorescence since they more rapidly undergo non-radiative Auger recombination. Consequently, the ESA 2 pathway that creates population on state-|2› should contribute little to the fluorescence quantum yield, and the value of Γ is expected to be comparatively small (Γ≈1) for fluorescence-detected 2D measurements. On the other hand, if the electron–hole pairs in the multiple exciton states become separated within a few picoseconds inside the photocell, the ESA 2 pathway should contribute to a significant photocurrent quantum yield, and the value of Γ is expected to be comparatively large (Γ≈2) for photocurrent-detected 2D experiments. Our model calculations show that this is indeed the case (see Supplementary Notes 1–3 , Supplementary Table 1 and Supplementary Figs 1–4 ). For low and high values of Γ, our simulated 2D spectra qualitatively resemble the fluorescence- and photocurrent-detected experimental data, respectively (see Fig. 5c,d ). Our results are in agreement with those of previous studies, in which efficient harvesting of charge carriers from MEG was observed in photocells [28] , [29] . Our results also have important implications for the general use of phase-modulation 2D spectroscopies that utilize an incoherent action signal, such as photocurrent or fluorescence. Such techniques provide selective spectroscopic information about the coherences and populations that contribute to the final observable, which can be important to understand how and which electronically excited material states are most relevant to the function of an optical or optoelectronic device. This approach holds promise to unravel the mechanistic details of the photophysical processes in a variety of material systems, and its advantages may benefit experiments that might otherwise be attempted using more conventional approaches to 2D electronic spectroscopy. Sample preparation of PbS colloidal QDs OLA-capped PbS QDs were prepared according to the procedure of Hines and Scholes [30] . PbS nanoparticles capped with the dithiol ligand sodium 2,3-DT were synthesized from OLA-capped nanoparticles by ligand exchange, as described previously [31] . The average core diameter was determined using transmission electron microscopy to be 3.6±0.6 nm. Solutions of nanoparticles were stored under air-free conditions until use. Fluorescence studies were performed with solutions of OLA-capped nanoparticles in toluene. The bandgap of these particles was determined from the absorption spectrum to be E g =1.1 eV. Photocell preparation Photoconductive cells were fabricated as previously described [31] . In brief, a concentrated (50 mg ml −1 ) solution of DT-capped PbS QDs in water was drop-casted onto lithographically designed interdigitated electrodes on glass slides that had been freshly cleaned using oxygen plasma. Drop casting and initial drying were performed in air, but the resulting samples were further dried and stored under vacuum. The electrodes consisted of 20 interdigitated Au fingers separated by 10–20 μm and a running length of 3 mm. The cells were biased at 5 V during photocurrent measurements using a potentiometer and the d.c. output of a Stanford Research SR570 current preamplifier. The resulting current was converted to a voltage signal using this same instrument. The QD photocell was maintained under vacuum during 2DPS measurements. Phase-modulation 2DPS We implemented phase-modulation 2DPS using a train of four collinear ultrafast laser pulses. The experimental set-up and laser pulse characteristics are very similar to those previously described for 2DFS performed at visible [15] , [16] , [17] , [19] and at ultraviolet wavelengths [18] . The phase-modulation method provides a means to isolate the fourth-order population contribution to the photocurrent signal, which is used to construct the 2D spectra. A 250-kHz pulse train is separated into four beams using two Mach–Zehnder interferometers. Within each Mach–Zehnder interferometer beam arm is placed an acousto-optic Bragg cell, which is used to impart a continuously varying phase-shift to each of the four laser pulses. The phases φ 1 , φ 2 , φ 3 and φ 4 associated with each of the four laser pulses, respectively, were modulated such that the relative phase between pulses 1 and 2 was set to φ 21 = φ 2 – φ 1 =5 kHz, and that between pulses 3 and 4 was set to φ 43 = φ 4 – φ 3 =8 kHz. The phase modulation of the pulse electric fields gives rise to a time-varying photocurrent signal at the ‘sum’ and ‘difference’ side-band frequencies φ 43 + φ 21 =13 kHz and φ 43 − φ 21 =3 kHz, respectively. Each of these non-linear signals scaled linearly with respect to the intenstities of pulses 1 and 2, and with respect to the intensities of pulses 3 and 4, so that the signal is proportional to the square of the total intensity. The two signals were simultaneously detected using two dual-channel lock-in amplifiers. The ‘sum’ and ‘difference’ signals correspond to the ‘non-rephasing’ and ‘rephasing’ response functions, respectively, which are often used in 2D spectroscopy [17] . The in-phase and in-quadrature (shifted by 90°) detection channels of the lock-in amplifiers provide the real and the imaginary parts of the response functions [15] . As described in the text, the 2D interferograms are collected as a function of the interpulse delays (designated as τ , T and t ) by varying the beam path lengths. The 2D response function S ( τ , T , t )is Fourier transformed with respect to the τ and t variables to obtain the 2D spectrum as a parametric function of the population period T . Computer calculations Computer simulations were performed using the QD model described in ref. 32 . The one-exciton band was modelled using two singly excited states with one resonant with the first two laser pulses, and the other corresponding to the ‘band edge’ state. The band edge state was used to calculate ESA signal contributions, where after the initial exciton population relaxes to the band edge, subsequent excitation to the two-exciton state is possible. Due to the many-body effects associated with the MEG on excitation using high energy photons, an EIS of 500 cm −1 was assumed. Within the framework of a line shape function-based description, broadening of the 2D line shape was taken into account due to the excitation induced electronic dephasing. For the simulations of the fluorescence-detected measurement, the value for Γ=1.1 was used. For the simulations of the photocurrent-detected measurement, the value for Γ=2 was used. For details of these calculations, see Supplementary Notes 1–3 , Supplementary Table 1 and Supplementary Figs 1–4 . How to cite this article: Karki, K. J. et al . Coherent two-dimensional photocurrent spectroscopy in a PbS quantum dot photocell. Nat. Commun. 5:5869 doi: 10.1038/ncomms6869 (2014).